Regenerative capacity in newts is not altered by repeated regeneration and ageing The extent to which adult newts retain regenerative capability remains one of the greatest unanswered questions in the regeneration field. Here we report a long-term lens regeneration project spanning 16 years that was undertaken to address this question. Over that time, the lens was removed 18 times from the same animals, and by the time of the last tissue collection, specimens were at least 30 years old. Regenerated lens tissues number 18 and number 17, from the last and the second to the last extraction, respectively, were analysed structurally and in terms of gene expression. Both exhibited structural properties identical to lenses from younger animals that had never experienced lens regeneration. Expression of mRNAs encoding key lens structural proteins or transcription factors was very similar to that of controls. Thus, contrary to the belief that regeneration becomes less efficient with time or repetition, repeated regeneration, even at old age, does not alter newt regenerative capacity. Newts are among vertebrates known to possess remarkable regenerative capacity of tissues, organs or body parts such as limbs, tails and eyes [1] . Because of these unparalleled regenerative deeds, newts could provide much coveted answers that regenerative medicine is presently seeking. Consequently, these animals have been the favoured models of regeneration research for over 200 years since discovery of these activities by Spallanzani in 1768 (refs 2 , 3 ). Significantly, regeneration in newts is mediated primarily by dedifferentiation or transdifferentiation of terminally differentiated cells. A fundamental and hitherto unanswered question regarding regeneration in these animals is whether regenerative ability declines with ageing or repetition of insult. This question has been difficult to answer because newts are wild animals (often of unknown age) and do not thrive in a laboratory setting. Spallanzani amputated limbs and tails from an animal (probably of larval stage, as he described them as young animals) six times over three months [2] . Also, as cited by Darwin, Bonnet performed a similar experiment eight times [4] . All of these experimenters concluded that repeated amputation led to limb regeneration but occasionally resulted in missing bone structures. However, it is unlikely that these experiments were well controlled: amputated limb stumps could have been exposed to the environment, introducing abnormalities. Also, the entire limb cannot be removed, because in such case no regeneration occurs [5] . To overcome these problems and address this important question, we have undertaken a long-term experiment on lens regeneration. Using our protocol, artificial incision of the cornea caused by lentectomy seals within one day, leaving the site of lens regeneration totally inside the eye. In addition, the lens is always removed in its entirety. Also, the lens regenerates from a different tissue, the pigment epithelial cells (PECs) of the dorsal iris, via transdifferentiation, rather than from remaining lens tissue [6] , [7] . In this study, we establish that lens regeneration, even after 18 rounds spanning 16 years remains robust, producing structurally normal lenses with normal gene expression as well. Our results indicate the repetition or age do not affect regenerative capabilities in newts. Morphology and gene expression in the regenerated lenses We succeeded in keeping Japanese newts Cynops pyrrhogaster alive for over 16 years after they were collected in 1994, during which time we removed the lens from the same animals 18 times (see Methods for the history of operations). We show that number 17 and number 18 regenerated lenses, obtained from the second-to-last and last experiments, respectively, are virtually identical to intact lenses removed from full-grown 14–year-old newts, produced from fertilized eggs (by G.E. and Y.E. ), which never underwent lens regeneration (Methods). Grossly, experimental and control lenses were of the same size and transparency. Lens fibre organization appeared remarkably normal with the nucleus containing primary fibres and the cortex containing secondary fibres ( Figs 1 and 2 ). Most importantly, we found that gene expression patterns were very similar in both groups. We used quantitative PCR (qPCR) to examine expression of crystallin genes, along with genes encoding transcription factors that regulate crystallin expression, such as Pax-6, Sox2, MafB, Sox1, Prox-1 and Delta, all of which function in lens development and lens fibre differentiation and are thus related to normal lens homeostasis. As can be seen in Figures 3 and 4 , gene expression levels show no statistically significant change between the two groups at P <0.05 ( t -test). Expression of all genes was normalized to that of two housekeeping genes, GAPDH and EF-1a . Regardless of the choice of housekeeping gene the results are very similar. mRNA expression levels between number 17 and number 18 were also similar. Only γ- crystallin appeared to be more highly expressed in number 18, but the difference was not significant at P <0.05 ( t -test). Overall, we conclude that repeated lentectomy does not alter the quality of the regenerated lens or perturb normal homeostasis. Our study also establishes that an animal's age is not a factor in regenerative capacity. As the newts were collected in the wild, it is impossible to know the exact age; however, on the basis of collecting experience and their relative size, we estimate these newts to have been at least 14-years-old when collected (Methods). Thus, by the end of the reported experiment, the animals are likely to be at least 30 years of age. It has been reported [8] that the lifespan of the Japanese newt is 25 years. However, wild newts collected in Obama, Fukui, Japan have been kept for over 30 years (G.E., unpublished observations), indicating that our newts are quite old and that they can live long if well cared for. 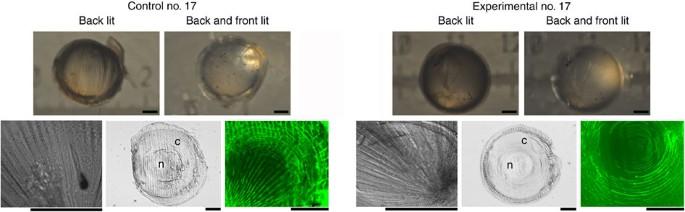Figure 1: Images of regenerated lenses after the seventeenth lentectomy. An experimental lentectomy no. 17 lens (right) compared with a control intact lens taken from an animal that had never undergone lens regeneration (control no. 17) (left). Top panels: photography of the whole lens (back lit or back and front lit). Note similarity in size and transparency as well as the normal arrangement of lens fibres around the equatorial circumference. Lower panels: sections from these lenses indicating a normal arrangement of lens fibres and normal lens morphology. From left to right: section showing lens fibre arrangement; a cross-section showing normal morphology of the lens with its nucleus (n) containing the primary fibres and the cortex (c) containing secondary fibres; staining of a section with β5-crystallin antibody to visualize fibres at higher magnification. Bar, 0.25 mm. Figure 1: Images of regenerated lenses after the seventeenth lentectomy. An experimental lentectomy no. 17 lens (right) compared with a control intact lens taken from an animal that had never undergone lens regeneration (control no. 17) (left). Top panels: photography of the whole lens (back lit or back and front lit). Note similarity in size and transparency as well as the normal arrangement of lens fibres around the equatorial circumference. Lower panels: sections from these lenses indicating a normal arrangement of lens fibres and normal lens morphology. From left to right: section showing lens fibre arrangement; a cross-section showing normal morphology of the lens with its nucleus (n) containing the primary fibres and the cortex (c) containing secondary fibres; staining of a section with β5-crystallin antibody to visualize fibres at higher magnification. Bar, 0.25 mm. 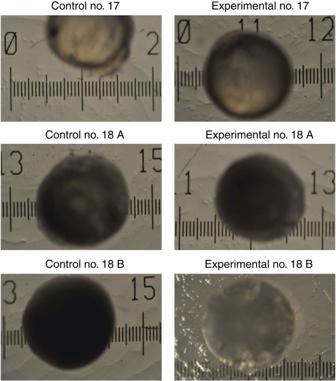Figure 2: Size of experimental and control regenerated lenses. Samples of regenerated lenses after the 17th (experimental no. 17) or the 18th (experimental no. 18) lentectomy compared with respective controls. Two samples from the eighteenth regeneration labelled as sample A and B are shown. Controls were intact lenses from animals that had never undergone regeneration. Images include a scale bar (a ruler with a basic unit of 1 mm) to indicate similarity in size of experimental and control lenses. Full size image Figure 2: Size of experimental and control regenerated lenses. Samples of regenerated lenses after the 17th (experimental no. 17) or the 18th (experimental no. 18) lentectomy compared with respective controls. Two samples from the eighteenth regeneration labelled as sample A and B are shown. Controls were intact lenses from animals that had never undergone regeneration. Images include a scale bar (a ruler with a basic unit of 1 mm) to indicate similarity in size of experimental and control lenses. 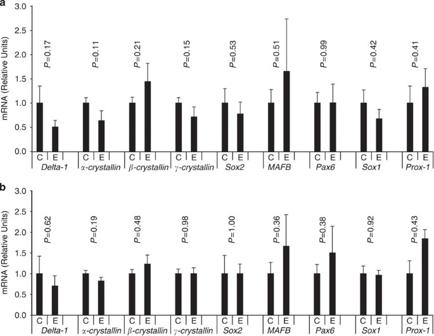Figure 3: qPCR analysis of gene expression after 17 lentectomies. Four different sets of lenses (from four different animals) were used and RNA was prepared separately from each. qPCR analysis was performed for each sample and the data combined, as shown in figure. C, control groups; E, experimental, no. 17. (a) qPCR data were normalized to housekeeping gene,GAPDH. (b) qPCR data were normalized to housekeeping geneEF1-a. Bars indicate the standard error of the mean (s.e.m.). Statistical analysis byt-test. Full size image Figure 3: qPCR analysis of gene expression after 17 lentectomies. Four different sets of lenses (from four different animals) were used and RNA was prepared separately from each. qPCR analysis was performed for each sample and the data combined, as shown in figure. C, control groups; E, experimental, no. 17. ( a ) qPCR data were normalized to housekeeping gene, GAPDH . ( b ) qPCR data were normalized to housekeeping gene EF1-a . Bars indicate the standard error of the mean (s.e.m.). Statistical analysis by t -test. 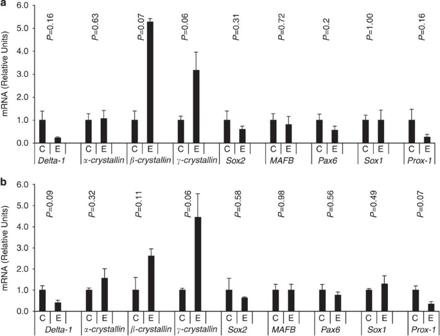Figure 4: qPCR analysis of gene expression after 18 lentectomies. Four different sets of lenses (from four different animals) were used and RNA was prepared separately from each. qPCR analysis was performed for each sample and the data combined, as shown in figure. C, control groups; E, experimental, no. 18. (a) qPCR data were normalized to housekeeping gene,GAPDH. (b) qPCR data were normalized to housekeeping geneEF1-a. Bars indicate the standard error of the mean (s.e.m.). Statistical analysis byt-test. Full size image Figure 4: qPCR analysis of gene expression after 18 lentectomies. Four different sets of lenses (from four different animals) were used and RNA was prepared separately from each. qPCR analysis was performed for each sample and the data combined, as shown in figure. C, control groups; E, experimental, no. 18. ( a ) qPCR data were normalized to housekeeping gene, GAPDH . ( b ) qPCR data were normalized to housekeeping gene EF1-a . Bars indicate the standard error of the mean (s.e.m.). Statistical analysis by t -test. Full size image General observation throughout the 16-year duration As we could not kill the animals during the 16-year period, the progress of regeneration as to rate or stages was evaluated carefully through detailed observation. We could not find any significant delay in the process of lens regeneration in all 18 repetitions. Each step, depigmentation, lens rudiment (lens vesicle) formation and so forth was within the regular period of time according to the stages defined by Sato [9] . For example, depigmentation at the dorsal marginal iris started from 7-to-10 days after lens removal, and lens vesicle formation was observed on day 10–14 after lens removal in all 18 times. In addition, no significant difference in the rate of differentiation and growth of the regenerating lens was documented. The regenerated lens attained normal size in diameter within 5 months after lens removal in all 18 experiments. Again, no significant change in growth rate was documented. Cataractous changes were never observed throughout the 18 repetitions of lens regeneration. All the regenerated lenses were completely transparent. Likewise, we carefully examined the isolated lens at the time of collection using a stereoscopic microscope. No structural abnormalities were ever documented. The discovery of lens regeneration by Collucci in 1891 (ref. 10 ) and independently by Wollf in 1895 (ref. 11 ) poses an important evolutionary question. Although regeneration of a partly injured eye was known for many years before the findings of Collucci and Wollf [12] , it was not until Darwin proposed his theory of evolution that scientists considered regeneration in an evolutionary context. Thus, Wollf proposed in 1894 that lens regeneration alone without eye injury must not confer a selective advantage, because removal of only the lens without eye injury does not occur naturally [13] . On the basis of this idea, he performed experiments leading to discovery of lens regeneration and concluded that potent regenerative capability must be conserved in this animal as 'Zweckmäessigkeit,' meaning effectiveness or usefulness for a certain procedure. This was also discussed at length by Morgan in 1901 (ref. 14 ) as an example of how the likelihood of regeneration is not correlated with the probability of injury. Our findings clearly indicate that this is the case. Because regeneration can be so constant after so many years, it suggests that regeneration is an attribute that is expressed by many organisms. Our observation that regenerative ability in newts does not decline with repetition or over time suggests that mechanisms that underlie these activities are not altered by the debilitating effects of injury and ageing. It is also possible that the newt might use novel mechanisms to protect its cells from harmful mutations that might be introduced over long periods of time. It is important that no cataract (a common disease of the lens related to ageing) was ever observed. Moreover, our observations have significant consequences on the role of 'precursor' cells for lens transdifferentiation. If the source of the regenerating lens is cells of the iris that do not replenish themselves, then, by the 18th time there would be hardly any iris left. To alleviate such a problem two possibilities can be considered. First, that loss of iris PECs results in regeneration of iris from precursor cells and thus there is source of cells all the time. Second, that as the PECs divide, both daughter cells do not contribute to transdifferentiation, as one of them should be maintained as a PEC. The latter possibility seems most probable as the same occurs during retina regeneration from the retina pigment epithelium. In this sense, somatic PECs behave as progenitor cells. Such patterns of proliferation have not been studied well in this system, and our present data provide the impetus to identify them. Also, based on the fact that carcinogens induce lens regeneration even from the ventral iris (but no cancer) [15] , [16] it is possible that signalling related to oncogenesis inhibits the action of replicative senescence during regeneration. In addition, despite beliefs that aged animals regenerate less efficiently than young ones (also discussed by Darwin [4] ), our experiments show that this is not the case in the newt. As regenerative medicine has entered a new era, the knowledge that aged tissues possess robust regenerative capabilities should provide the impetus to identify mechanisms underlying this capacity in the newt and compare them with strategies being employed to promote mammalian regeneration, such as the creation of iPS cells. Our findings, thus, are of paramount importance to the field of regeneration and ageing. Animals and operations Adult male newts Cynops pyrrhogaster were collected in Okazaki, Japan in 1994. At the time, we estimate that they were at least 14 years of age: one of us (G.E., unpublished observations) has determined that it takes more than 14 years for the body of a male newt to attain 90% the size of a full-grown newt (average body length: 11.6±2 cm). When collected the average body length of our specimens was equivalent to that of full-grown male newts. Thus by the end of our experiments these animals were likely almost 30 years old. The first fourteen lentectomies were performed every April 15 and October 15 from 1996 to 2002. Lentectomies number 15 and number 16 were performed on the same dates in 2008. Lentectomies number 17 and number 18, which provided tissues for this analysis were performed on July 9, 2009 and February 2, 2010, respectively. Lenses from newts of similar size that had never been lentectomized served as controls. Control newts were born in 1996 from eggs collected in the laboratory, and at the time of lens collection for RNA analysis, they were about 14-years-old. Usage of animals complied with the institutional regulations. For lentectomies, newts were anaesthetized in 0.1% ethyl 3-aminobenzoate (Sigma) prepared in fresh water. Using a sharp blade, an incision was made in the cornea along the nasal temporal axis. The lens was then removed in its entirety with fine forceps. Histology and immunofluorescence Whole lenses were fixed and kept in 1% PFA. After paraffin embedding and before sectioning, tissue blocks were soaked in cold water, allowing the lens to soften and improving tissue morphology. 10 μm sections were stained with mouse β5-crystallin antibody to visualize lens fibre arrangement. RNA isolation reverse transcription and first-strand cDNA synthesis Total RNA was extracted from carefully isolated regenerated lenses after lentectomy using the Qiagen RNeasy Plus purification kit (Qiagen). Samples were then flash-frozen in liquid nitrogen and homogenized using lysis buffer from the kit, and RNA isolation was performed according to the manufacturer's instructions. Briefly, samples were lysed and homogenized in a highly denaturing guanidine-isothiocyanate–containing buffer. The lysate is then passed through a gDNA eliminator spin column to remove genomic DNA. Ethanol is added to the flow-through to provide appropriate binding conditions for RNA, and the sample is then applied to an RNeasy spin column, where total RNA binds to the membrane and contaminants are washed away. High-quality RNA is then eluted in 30 μl, or more, of water. Quantities of 100 ng of total RNA were reverse transcribed using Invitrogen Superscript II reverse transcriptase according to the manufacturer's instructions (Invitrogen). First-strand complimentary DNA synthesis was performed using SuperScript II RT. Quantitative PCR Quantitative PCR was performed using a Stratagene MX300 machine (Agilent). The SYBR GreenER (Invitrogen) qPCR reagent system was used to amplify cDNA. The following primers were: Gapdh forward, 5′-GCATGCTGTGACTGCTACACAAAAG-3′ and reverse, 5′-GCTGGAATGATATTCTGGTTTGCAC-3′; Ef1a forward, 5′-GCACCACGAGGCGCTGGT-3′ and reverse, 5′-CAACACAGGAGCGTATCCCTG-3′; alphaA-Crystallin forward, 5′-TCACCGGAAGACCTAAGTGTC-3′ and reverse, 5′-GGTCAGCATGCCATCAGTGG-3′; betaB1-Crystallin forward, 5′-GGATACCTGGTCTAACAG-3′ and reverse, 5′-GCCACTGCATGTCCCTG-3′; gamma-Crystallin forward, 5′-CCTATGAGTGCAGCACTGAGT-3′ and reverse, 5′-GTCATTGAAGCCCATCCAGTG-3′; Delta1 forward, 5′-CCGACCGGCTCATCAGTCGT-3′ and reverse, 5′-CCCCGCAGGTGAAGTGCC-3′; Mafb forward, 5′-AGAGCACCACGCCTCGGA-3′ and reverse, 5′-GACAATCCCCAACACAAC-3′; Pax6 forward, 5′-AGGCCTCCTCCTACTCTTGC-3′ and reverse, 5′-GGGAAATGAGACCTGTCGAA-3′; Prox1 forward, 5′-ACATGTGCAGCAACTCTTCG-3′ and reverse, 5′-CATCCCTCGGATGATGTTCT-3′; Sox1 forward, 5′-CGCCCTGTCCGCAGAGG-3′ and reverse, 5′-GCTAGGATAGCCGCATGTTC-3′; and Sox2 forward, 5′-AAGTTTCGCCAACTTCC-3′ and reverse, 5′-GGAGTTAAGAATGCCGGTG-3′. Steps used to perform qPCR analysis included a hold step at 50 °C for 2 min to activate uracil-DNA glycosylase, followed by another hold at 95 °C for 10 min. Samples then underwent 38 cycles of 95 °C for 30 s followed by 58–60 °C for 45 s. Subsequently, melt analysis was performed by increasing the temperature from 65 to 95 °C. Relative expression levels were calculated using the ΔΔ C t -method in which the d C t value for each gene was first calculated by subtracting the C t value (lowest) of a sample from rest of the samples C t values. Then the Relative Unit (RU) was calculated as log2 of the C t value. RU values of all genes were then normalized to the RU value of the housekeeping gene (EF1a or GAPDH) for each sample by dividing the RU of a sample with that of the corresponding housekeeping gene. Average RUs from four control and four experimental samples were then calculated and plotted in individual graphs. A t -test was used to calculate P -values for significance. How to cite this article: Eguchi, G. et al . Regenerative capacity in newts is not altered by repeated regeneration and ageing. Nat. Commun. 2:384 doi: 10.1038/ncomms1389 (2011).